Integrating sequence and array data to create an improved 1000 Genomes Project haplotype reference panel A major use of the 1000 Genomes Project (1000GP) data is genotype imputation in genome-wide association studies (GWAS). Here we develop a method to estimate haplotypes from low-coverage sequencing data that can take advantage of single-nucleotide polymorphism (SNP) microarray genotypes on the same samples. First the SNP array data are phased to build a backbone (or ‘scaffold’) of haplotypes across each chromosome. We then phase the sequence data ‘onto’ this haplotype scaffold. This approach can take advantage of relatedness between sequenced and non-sequenced samples to improve accuracy. We use this method to create a new 1000GP haplotype reference set for use by the human genetic community. Using a set of validation genotypes at SNP and bi-allelic indels we show that these haplotypes have lower genotype discordance and improved imputation performance into downstream GWAS samples, especially at low-frequency variants. Over the last few years the use of next generation sequencing technologies has lead to new insights in both population and disease genetics, by providing a more complete characterization of DNA sequences than is possible using genome-wide micro arrays. However, high coverage sequencing in large cohorts is still prohibitively expensive, and an experimental design involving low-coverage sequencing has become popular. For example, the 1000 Genomes Project (1000GP) is using 4 × coverage sequencing of ~\n2,500 samples from a diverse set of worldwide populations [1] . A consequence of the low-coverage sequencing is that some genotypes are only partially observed, and directly calling genotypes one site at a time can lead to low-quality call rates [2] . The current paradigm for detecting, genotyping and phasing polymorphic sites from low-coverage sequence data starts by mapping sequence reads to a reference genome. Mapped reads that overlap a given site in a single individual are then combined together to form genotype likelihoods (GLs). Genotype likelihoods are the probabilities of observing the reads given the underlying (unknown) genotypes at each site. Improved call rates can be achieved by aggregating information across many samples through the use of phasing methods that estimate the underlying haplotypes of the study samples. Inference of the underlying haplotypes dictates the genotype calls of each sample. This builds on the idea that over small genomic regions, the samples will share haplotypes due to local genealogical relationships, leading to a per-haplotype coverage much higher than the per-individual coverage. To achieve this haplotype phasing and genotype calling, the hidden Markov model (HMM)-based phasing methods that were primarily designed to estimate haplotypes from single-nucleotide polymorphism (SNP) array data were adapted to deal with sequencing data. For example, the 1000GP phase 1 set of haplotypes from 1,092 individuals was estimated using a combination of Beagle [3] and MaCH/Thunder [4] . Such haplotype reference panels are now routinely used to impute unobserved genotypes in genome-wide association studies (GWAS), as this increases power to detect and resolve associated variants and facilitates meta-analysis [5] . Our recent research suggests that the SHAPEIT2 method is currently the most accurate method for phasing sets of known genotypes. The method uses a similar HMM to approaches such as Impute2 (ref. 6 ) and MaCH. A key feature of the method is that the HMM calculations are linear in the number of haplotypes being estimated, whereas Impute2 and MaCH scale quadratically. The method uses a unique approach that represents the space of all possible haplotypes consistent with an individual’s genotype data in a graphical model. A pair of haplotypes consistent with an individual’s genotypes are represented as a pair of paths through this graph, with constraints to ensure consistency that are easy to apply due to the model structure. For this reason SHAPEIT2 is among the most computationally tractable methods [7] , [8] . Here we present a new version of SHAPEIT2 that estimates haplotypes from GLs generated by low-coverage sequencing data. In addition, our new method can also take advantage of SNP microarray genotypes on the same samples. The majority of the ~\n2,500 1000GP sequenced samples have been genotyped on either the Illumina Omni 2.5 or Affymetrix 6.0 microarray, as well as an additional set of 1,198 unsequenced samples, many of whom are close relatives of the ~\n2,500 sequenced samples. Our overall approach has two steps: first the SNP array data are phased to build a backbone of haplotypes across each chromosome, which we refer to as the scaffold. Second, we take GL data at sequenced variant sites, and jointly phase this data ‘onto’ this haplotype scaffold. The first advantage of this approach is that the relatedness between the extended set of genotyped samples leads to a very accurate phased scaffold. For the analysis in the paper, this set included 392 mother–father–child trios, 30 parent–child duos and 905 nominally unrelated samples. The phasing of trios and duos is expected to be highly accurate due to the Mendelian constraints on the underlying haplotypes. The phasing of the unrelated samples will benefit from being phased together with these trios and duos. The second advantage is that the phasing of the GL data onto the scaffold is carried out in chunks. As the variants in each region are phased ‘onto’ the scaffold, no further work is needed to combine the regions together. As such, the method is highly parallelizable. This approach generalizes our MVNcall [9] , approach which is designed to phase one variant site at a time onto a haplotype scaffold, and improves upon its accuracy, by phasing multiple sites jointly onto the scaffold and using a more sophisticated underlying model. Our method is unique in its ability to phase GL data at multiple sites jointly, together with a phased scaffold at a subset of sites. Methods such as Beagle [3] and MaCH/Thunder [4] could be made to accept a scaffold of unphased genotypes, by recoding the genotypes as sequenced variants at very high coverage. However, our two-stage approach allows valuable family information to be used in phasing the scaffold. To demonstrate the benefits of this new method, we applied it to the 1000GP phase 1 sequence data to produce new haplotypes. We then compared these haplotypes with the existing set of 1000GP phase 1 haplotypes, and also to a set of haplotypes produced by Beagle. In all the experiments, we used the set of GLs available on the FTP website for 1,092 phase 1 samples. These consist of GLs at 36,820,992 SNPs, 1,384,273 bi-allelic indels and 14,017 structural variations (SVs). To create the haplotype scaffold (Omni 2.5 M), we used Illumina Omni 2.5 genotypes available on 2,141 samples and 2,368,234 SNPs. We phased this data set using the existing version of SHAPEIT2 (r644). 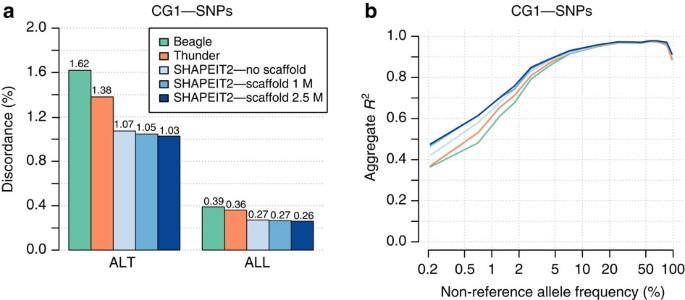Figure 1: Methods comparison of genotype discordance and imputation accuracy using the CG1 data. (a) Shows the discordance at chr20 CG1 SNP genotypes of Beagle (green), Thunder (orange) and SHAPEIT2 without using a scaffold (light blue), using a 1 M SNPs haplotype scaffold (medium blue) and using a 2.5 M SNPs haplotype scaffold (dark blue). ALT stands for the discordance at genotypes involving at least one non-reference allele, and ALL for the overall discordance. (b) Shows the performance of the previous call sets when used as a reference panel to impute four CG1 European samples genotyped on Illumina 1 M SNP array. Thexaxis shows the non-reference allele frequency of the SNP being imputed. Theyaxis shows imputation accuracy measure by aggregateR2. Supplementary Table 1 shows the number of trios, duos and unrelated samples in each of the 14 populations. To mimic the use of a sparser haplotype scaffold, we also created a new scaffold by thinning the Omni scaffold down to 1,000,000 SNPs (1 M). We then phased the GL data set on chromosome 20 in three different ways using (a) the Omni 2.5 M scaffold, (b) the 1 M scaffold, (c) no scaffold. We evaluated the quality of the different sets of haplotypes by looking at the concordance of the inferred genotypes to validation sets of SNP and indel genotypes. We used two validation data sets derived from Complete Genomics (CG) sequencing: a set of publicly available genotypes on 69 samples (CG1), and a larger set of 250 individuals sequenced for the purposes of 1000GP validation (CG2). Both of these data sets contain accurate genotypes that were derived from high coverage (~\n80 ×), and show enough overlap in variants and samples with phase 1 for relevant genotype discordance analysis. Supplementary Tables 2 and 3 show the overlap between the CG and 1000GP data sets in terms of samples and variant sites, respectively. Figure 1a shows the genotype discordance at CG1 SNPs. We measure discordance using just the validation genotypes that contain at least one copy of the non-reference allele (ALT) and all validation genotypes (ALL). These results show that the three haplotype sets produced by SHAPEIT2 (blue bars) have lower levels of discordance compared with Beagle haplotypes (green) and the 1000GP haplotypes (orange). For example, the CG1 ALT discordance of the SHAPEIT2 haplotypes made using the Omni 2.5 scaffold, and the ALT discordance of the 1000GP haplotypes, are 1.03 and 1.38%, respectively. In addition, we observe that the Omni 2.5 scaffold produced better results than the 1 M scaffold, which is in turn better than using no scaffold. 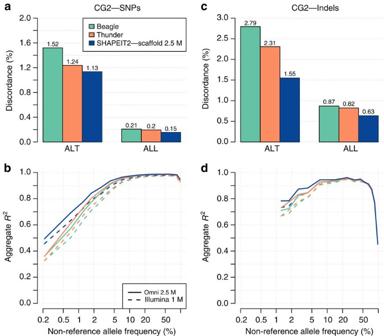Figure 2: Methods comparison of genotype discordance and imputation accuracy using the CG2 data. (a) Shows the whole genome genotype discordance of Beagle (green), Thunder (orange) and SHAPEIT2 using a 2.5 M SNPs haplotype scaffold (dark blue) at CG2 SNPs. (b) Shows the performance of the three call sets to impute SNPs on chromosome 10 in 10 CG2 European samples typed on Illumina 1 M and Omni 2.5 M chips. Thexaxis shows the non-reference allele frequency of the SNP being imputed. Theyaxis shows imputation accuracy measure by aggregateR2. (c) and (d) show similar results thanaandb, respectively for short bi-allelic indels instead of SNPs. Figure 2a,b shows the genotype discordance at CG2 SNPs and indels, where we observe the same pattern of performance between methods. We also find that this pattern holds across different ancestries ( Supplementary Fig. 1 ). The discordance on indels is worse than on SNPs ( Fig. 2c ). A reason for this difference may be that it is more challenging to map sequencing reads that contain indels, so the GLs for indels may be less informative than GLs at SNPs. Figure 1: Methods comparison of genotype discordance and imputation accuracy using the CG1 data. ( a ) Shows the discordance at chr20 CG1 SNP genotypes of Beagle (green), Thunder (orange) and SHAPEIT2 without using a scaffold (light blue), using a 1 M SNPs haplotype scaffold (medium blue) and using a 2.5 M SNPs haplotype scaffold (dark blue). ALT stands for the discordance at genotypes involving at least one non-reference allele, and ALL for the overall discordance. ( b ) Shows the performance of the previous call sets when used as a reference panel to impute four CG1 European samples genotyped on Illumina 1 M SNP array. The x axis shows the non-reference allele frequency of the SNP being imputed. The y axis shows imputation accuracy measure by aggregate R 2 . Full size image Figure 2: Methods comparison of genotype discordance and imputation accuracy using the CG2 data. ( a ) Shows the whole genome genotype discordance of Beagle (green), Thunder (orange) and SHAPEIT2 using a 2.5 M SNPs haplotype scaffold (dark blue) at CG2 SNPs. ( b ) Shows the performance of the three call sets to impute SNPs on chromosome 10 in 10 CG2 European samples typed on Illumina 1 M and Omni 2.5 M chips. The x axis shows the non-reference allele frequency of the SNP being imputed. The y axis shows imputation accuracy measure by aggregate R 2 . ( c ) and ( d ) show similar results than a and b , respectively for short bi-allelic indels instead of SNPs. Full size image We also used the CG samples not included in phase 1 to assess the quality of the estimated haplotypes when used as a reference panel for GWAS imputation [5] , [10] . We divided the CG1 sites into those on the Illumina 1 M SNP array, and then used these together with the different haplotype sets to impute the CG1 genotypes not on the array. We then measured the imputation accuracy against the CG1 genotypes. In the same way as previous evaluations [1] , we stratified SNPs and indels by their non-reference allele frequency in the 1000GP haplotypes so that each site is always assigned to the same frequency bin in the results. For each SNP or indel, we measured the R 2 of the imputed dosage estimates with the validation genotypes. Figure 1b plots the non-reference allele frequency versus R 2 and shows that the use of a haplotype scaffold clearly leads to an increase in R 2 especially at lower frequencies. For example, at 0.5% frequency, the SHAPEIT2 haplotypes made with a 2.5 M scaffold increase R 2 by 0.1 compared with the 1000GP phase 1 set of haplotypes. We also find that using the 1 M scaffold produces almost identical imputation performance to the 2.5 M scaffold. Running SHAPEIT2 without a scaffold produces results intermediate to those of the scaffolded haplotypes and the 1000GP phase 1 set of haplotypes. Figure 2c,d shows the imputation performance of SNPs and indels, respectively when using the CG2 validation set. For this experiment we carried out imputation using genotypes on the Illumina 1 M and Omni 2.5 M chip. We also observe that SHAPEIT2 haplotypes using the 2.5 M scaffold produce improved imputation performance compared with the 1000GP phase 1 set of haplotypes and the Beagle haplotypes, again independently of the sample ancestry ( Supplementary Fig. 2 ). As expected, using a denser chip the imputation improves the results. At 1% frequency SNPs, we find that the imputation from the SHAPEIT2 scaffold reference haplotypes into genotypes on the Omni 2.5 M chip and the Illumina 1 M chip produce R 2 measures of 0.78 and 0.73, respectively. Interestingly, imputation from the 1000GP phase 1 set of haplotypes into genotypes on the Omni 2.5 M chip produces an R 2 =0.73. This highlights the value of using a scaffolded set of haplotypes. In terms of imputation performance, the value of using a scaffold set of haplotypes is equivalent to the use of a much denser SNP chip in the GWAS samples. The indel imputation results in Fig. 2d show some differences to the SNP imputation results at high frequencies, but are otherwise broadly similar. We investigated this issue and discovered that indels within 50 bp of another indel had noticeable lower imputation accuracy than more isolated indels. 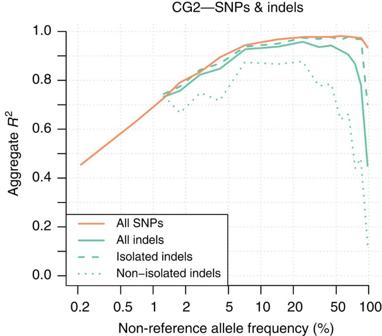Figure 3: Imputation accuracy at SNPs and indels using the CG2 data. The imputation performance at SNPs and indels are shown with the orange and green lines, respectively. Performance at all indels, isolated indels and non-isolated indels are shown using plain, dashed and dotted lines. An indel is isolated when no other indels is in the 50 bp flanking regions. Thexaxis shows the non-reference allele frequency of the SNP being imputed. Theyaxis shows imputation accuracy measure by aggregateR2. Figure 3 shows the imputation performance of indels stratified by distance to another indel, together with the SNP imputation results. This figure shows that isolated indels can be imputed with very similar levels of accuracy to SNPs. Figure 3: Imputation accuracy at SNPs and indels using the CG2 data. The imputation performance at SNPs and indels are shown with the orange and green lines, respectively. Performance at all indels, isolated indels and non-isolated indels are shown using plain, dashed and dotted lines. An indel is isolated when no other indels is in the 50 bp flanking regions. The x axis shows the non-reference allele frequency of the SNP being imputed. The y axis shows imputation accuracy measure by aggregate R 2 . Full size image Over the past year, the 1000 Genomes phase 1 haplotypes have been extensively used in many genetic studies, most of the time as reference panel to carry out GWAS imputation. In this paper, we showed that using the SHAPEIT2 phasing model, and integrating phased SNP array data, produces more accurate genotype and haplotype estimates. Using the resulting haplotypes as reference panel for GWAS imputation provides better prediction of untyped variants at rare SNPs and indels across a range of ancestries and SNP arrays. This highlights the potential of using this new set of haplotypes in future GWAS studies. The new haplotype reference set is available from the website ftp://ftp.1000genomes.ebi.ac.uk/vol1/ftp/phase1/analysis_results/shapeit2_phased_haplotypes/ and our new methods are available from the website http://www.stats.ox.ac.uk/?marchini/#software . We expect that many other studies may be able to make use of our approach to produce highly accurate haplotypes in their samples. It is likely that many cohorts that undergo sequencing will already have SNP microarray genotypes available. For example, twin studies that have sequenced one individual from each dizygotic twin pair, and also have genotype data on all individuals, may benefit substantially from using our approach. The phasing of the twins genotype data will be highly accurate in regions of shared haplotypes, and this will help in genotype calling and phasing of the sequence data. Studies which have sequenced one individual from parent–child pairs will benefit in a similar manner. The final version of the 1000GP haplotypes on all of the ~\n2,500 samples will be phased using our new approach. We predict that further advances in haplotype accuracy are possible. First, it has recently been shown by ourselves and others that leveraging phase information in sequencing reads can lead to improved genotype calls and haplotype sets with lower switch error. In parallel work [11] , we have extended SHAPEIT2 to utilize phase informative reads after genotypes have been called, and have shown that this improves phasing accuracy. Other authors [12] , [13] have recently shown that joint inference of genotypes and haplotypes can improve both genotype and haplotype calls. However, it is yet to be determined how such improvements translate into downstream imputation accuracy. It is more likely that downstream imputation accuracy can be improved by increasing sample size of the reference panel. Efforts are now under way to create larger sets of haplotypes by combining together many low-coverage sequencing studies http://www.haplotype-reference-consortium.org/ . The phasing model for low-coverage sequence data We wish to estimate the haplotypes of N unrelated individuals with sequence data at L bi-allelic variants, which could be either SNPs, indels or structural variants. Our new algorithm extends the SHAPEIT2 model and the Markov chain Monte Carlo (MCMC) method used to carry out inference from this model. We use a Gibbs sampling scheme in which each individual’s haplotypes are sampled conditional upon the sequence reads of the individual and the current estimates of all the other individuals. Thus it is sufficient for us to consider the details of a single iteration in which we update the haplotypes of the i th individual. We use R to denote the sequence data available for this individual and H to denote the current haplotype estimates of other individuals being used in the iteration. We define the genotype likelihood as the probability of observing the sequence data R at a particular site l given the unobserved genotype G l : P ( R | G l ), where G l =0, 1, 2 counts the number of non-reference alleles in the genotype. These GLs can be obtained using specialised software like SAMtools [14] , SNPtools [15] or GATK [16] that derive these likelihoods directly from the BAM files containing the sequence reads. In each iteration we must sample a pair of haplotypes ( h 1 , h 2 ) for the i th individuals given both R and H . To do so, we adapted the parsimonious representation of the possible haplotypes of SHAPEIT to deal with GLs. We divide the region being phased into a number, C , of consecutive non-overlapping segments such that each segment contains eight possible haplotypes consistent with the GLs. In the case of bi-allelic variants, it means that each segment spans three sites, and we will see in the next section how this number can be increased. We use S l ε{1,…, C } to denote the segment that contains the l th SNP and b s and e s to denote the first site and the last site included in the s th segment, respectively. We use A lb to denote the allele carried at the l th site by the b th consistent haplotype. We can now represent a possible haplotype as a vector of labels X ={ X 1 ,…, X L } where X l denotes the label of the haplotype at the l th site in the S l th segment. The segmentation implies that the labels are identical within each segment so that we always have X l = X l −1 when S l = S l −1 . We use X { s } to define the label of the haplotype across all sites residing in the s th segment. Moreover, we represent a pair of haplotypes as a pair of vectors of labels ( X 1 , X 2 ). An illustration of this graph representation of the possible haplotypes can be seen in Supplementary Fig. 3a . Given the segment representation described above, sampling a diplotype (pair of haplotypes) given a set of known haplotypes H and a set of sequencing reads R involves sampling from the posterior distribution Pr ( X 1 , X 2 | H , R ). By assuming first that the reads for the individual we are updating, R , are conditionally independent of the haplotypes in other individuals, H , given the pair of haplotypes ( X 1 , X 2 ) we can write This factorization involves a model of the diplotype given the observed haplotypes, P ( X 1 , X 2 | H ) and for this we use the previously described SHAPEIT2 model [8] . The term P ( R | X 1 , X 2 ) is constructed from the GLs. On the basis of the segmentation of the chromosome into C segments, we employ a similar Markov model as the one introduced in the SHAPEIT2 method [8] . It can be written as: The idea here is to sample first a diplotype for the first segment s =1 from and then for each successive segment from . The scheme we use is described by the following steps: 1. A pair of haplotypes in the first segment with labels ( i , j ) is sampled with probability proportional to . 2. While s ≤ C a pair of haplotypes ( d , f ) for the s th segment is sampled given the previously sampled pair ( i , j ) for the { s −1}th segment with probability proportional to . 3. Set s = s +1. 4. If s = C +1 then stop, else go to step 2. The result is a pair of vectors of haplotype labels, X 1 and X 2 , across the whole region being phased and these can be turned into new haplotype estimates, ( h 1 , h 2 ), using for i ε{1, 2}. These haplotype estimates can then be added back into the haplotype set H and the next individual’s haplotypes can be estimated, although their current haplotype estimates must be removed from H first. To carry out this Markov-based sampling, we need now to describe how to obtain the two distributions and . To do so, we decompose them by using equations (1) and (2) as follows: We use the SHAPEIT2 model for the terms and . We do not give more details here since a complete description can be found in the SHAPEIT2 paper [8] . The GLs enter the model in the term P ( R | X 1 , X 2 ) as a product over all L sites as which implies that Initialization and MCMC iterations The experience of the 1000GP analysis group is that phasing approaches based on HMMs such as Thunder and Impute2 are slow to converge when applied to low-coverage sequence data if the starting haplotype estimates are initialized randomly. It has been observed that the Beagle method does not have this property, and that Thunder and Impute2 benefit from using an initial set of haplotypes estimated via Beagle. The 1000GP phase 1 haplotypes were estimated in this way by first running Beagle and then using these haplotypes as initial estimates in the Thunder model [1] . We initialize some of the genotypes by using the genotype posteriors P ( G l | H , R ) provided by the Beagle phasing model. Our approach relies on fixing the genotypes with high posterior probabilities and then use our model to call all the remaining genotypes ( Supplementary Fig. 3b ). Fixing highly confident genotypes is beneficial as it implies additional constraints on the space of possible haplotypes. In practice, segments then tend to contain more sites than in the default model: 32 sites on average per segment when applied to 1000GP instead of only three sites if no genotypes are fixed. We empirically determined a threshold on the Beagle posteriors to fix genotypes while maintaining relatively low discordance rates. This approach relies on the Beagle posteriors being well calibrated. To do so, we defined a set of 23 different threshold values ranging from 0.5 to 0.999 and measured for each (1) the discordance between CG1 and genotypes with a posterior above the threshold and (2) the percentage of genotypes with posteriors falling below the threshold ( Supplementary Fig. 4a,b ). In addition, we also measured the proportion of discordances of the full Beagle call set falling below each threshold value ( Supplementary Fig. 4c,d ). From this experiment, we empirically determined that a threshold value of 0.995 gives good performance: it implies that around 97% of the genotypes can be directly fixed while maintaining a discordance against CG1 of 0.07% overall (ALL) and of 0.25% at genotypes involving at least one alternative allele (ALT). We find that the 3% of the genotypes that we choose not to fix contain over 80% of the genotypes found to be discordant. Thus it makes sense that these are the genotypes that we try to improve upon using our model. Our algorithm starts from the haplotype estimates produced by Beagle and then, each MCMC iteration consists of updating the haplotypes of each sample conditional upon a set of other haplotypes using the Markov model described in section A. Our algorithm for GLs follows an iteration scheme quite different than in the SHAPEIT2 algorithm described in Delaneau et al. (2012). Specifically, we carry out several stages of pruning and merging iterations, instead of a single set of pruning and merging. In practice, we use 12 stages of four iterations (=48 iterations). We do not use burn-in iterations as we already have an initial estimate provided by Beagle. Each pruning and merging stage is used to remove unlikely states and transitions from the Markov model that describes the space of haplotypes with each individual. When enough transitions are pruned we merge adjacent segments together. This has the effect of simplifying the space of possible haplotypes so that a final set of sampling iterations can be carried out more efficiently. In practice, as we multiply these pruning and merging stages, the size of the model (that is, the graphs) tend to converge as shown by the evolutions of the number of sites per segment ( Supplementary Fig. 5a ) and the total number of segments ( Supplementary Fig. 5b ). Finally, to complete the model, we only use a subset of all available haplotypes when updating each individual as done in SHAPEIT2. We used a carefully chosen subset containing K 1 =400 haplotypes that most closely match the haplotypes of the individual being updated [10] . Note that the haplotype matching is carried out on overlapping windows of size W =0.1 Mb. Moreover, we also found useful to use an additional set of K 2 =200 randomly chosen haplotypes to help the mixing of the MCMC. So in total, we used K =600 conditioning haplotypes. Using such a large number of conditioning haplotypes is facilitated as SHAPEIT2 has linear complexity with K . Using a haplotype scaffold We denote as F the pair of haplotypes derived from SNP array for the i th individual, now the goal is to sample a pair of haplotypes from P ( X 1 , X 2 | H , R , F ) such that they are fully consistent with F . The scaffold F imposes a set of hard constraints on the space of possible haplotypes generated by the sampling scheme as illustrated in Supplementary Fig. 3c . So in the first segment when the pair of haplotypes defined by is fully consistent with F over the first segment, and 0 otherwise. Similarly, we define when the haplotype pair defined by is fully consistent with F over the segments s and s −1, and 0 otherwise. In practice, setting some of the transition probabilities that are inconsistent with F to 0 between successive segments means that it becomes impossible to sample haplotypes inconsistent with F across the full set of L sites. 1000GP phase 1 low-coverage sequence data We downloaded the GLs for 1,092 1000GP samples from ftp://ftp.1000genomes.ebi.ac.uk/vol1/ftp/release/20110521/ . This data set contains GLs for 36,820,992 SNPs, 1,384,273 short bi-allelic indels and 14,017 SVs. The GLs for SNPs were computed using SNPtools [15] , for indels using (ref. 16 ) and SVs using (ref. 17 ). We ran Beagle and SHAPEIT2 on the whole genome in chunks of 1.4 Mb with 0.2 Mb overlaps between flanking chunks. Beagle was run using 20 iterations instead of the 10 by default, otherwise, all other default settings were used. SHAPEIT2 was run using 78 iterations: 12 stages of 4 pruning iterations plus 30 main iterations. The estimation was carried out in windows of size W =0.1 Mb, using k =600 conditioning haplotypes; 400 chosen by Hamming distance and 200 chosen at random. All these computations were done using an ~\n1,000 CPU nodes cluster. SHAPEIT2 and Beagle required ~\n289 and ~\n99 CPU months, respectively to phase the whole genome 1000GP phase 1 data set. The multi-threading property of SHAPEIT2 proved to be very convenient on clusters with low memory nodes (for example, only 2–3 Gb of RAM per CPU core). For instance, on a single 8 CPU node, it is much more memory efficient to phase with SHAPEIT2 eight chunks of data sequentially each using eight threads than running the eight chunks in parallel. Both strategies need roughly the same running times whereas the second requires sharing of memory between the eight chunks. 1000GP Illumina Omni 2.5 SNP array data For the haplotype scaffold, we used a set of 2,141 samples genotyped on Illumina Omni 2.5 M. This set of samples includes all the 1000GP phase 1 samples. This data set contains some parent–child duos and mother–father–child trios, and in some cases just a subset of each family has been sequenced. Supplementary Table 1 gives details of sequenced and non-sequenced samples. We found that 380 and 30 phase 1 1000GP sequenced samples are part of trios and duos in this data set. SNPs with a missing data rate above 10% and a Mendel error rate above 5% were removed, leaving a total of 2,368,234 SNPs ready for phasing. We phased this data using SHAPEIT2 (r644) using all default settings ( W =2 Mb, K =100 haplotypes, iterations=45) and using all available family information. We used the resulting haplotypes as a scaffold to call the variant sites in 1000GP. The whole genome overlap between both data sets contains 2,183,314 SNPs. Complete Genomics (CG) validation data As validation data, we used two different data sets: the 69 genomes from Complete Genomics (CG1) and an additional set of 250 samples (CG2) also sequenced by CG. All these samples were sequenced using the Complete Genomics sequencing technology at an average of 80 ×. The CG1 can be found at http://www.completegenomics.com/public-data/69-Genomes/ and the CG2 at ftp://ftp.1000genomes.ebi.ac.uk/vol1/ftp/technical/working/20130524_cgi_combined_calls/ . On these data sets, we filtered out all variants with a call rate below 66% and ignored them in all posterior validation analysis. In both the data sets, we used called SNPs as validations. We found 15,060,295 and 17,399,956 1000GP SNPs overlapping CG1 and CG2, respectively. In addition, we found 554,886 1000GP indels also in CG2. In terms of sample overlap with 1000GP, CG1 and CG2 contain 34 and 125 samples, respectively. We used genotypes of these samples to measure discordance with the 1000GP call sets. As CG genotypes were derived from an average coverage of 80 × , we assume that they are accurate and thus can be considered as the truth in the validation process. We define the discordance as being the percentage of these CG genotypes that are miscalled by a software (Beagle, Thunder or SHAPEIT). We measure both the overall (ALL) discordance and the discordance at genotypes with at least one non-reference allele (ALT). In all discordance measures, we systematically exclude all genotypes at SNPs included in the Omni 2.5 M chips. We also used CG samples that are not in 1000GP nor related with any samples in 1000GP to assess the performance of the various call sets when used as reference panels for imputation. In CG1, we found 20 such samples, and 51 in CG2. To mimic a standard GWAS, we extracted genotypes at subsets of SNPs in both the data sets: for CG1, at all SNPs on chromosome 20 also included in the Illumina 1 M chip for CG1 (set A), and for CG2, at all SNPs on chromosome 10 also included in the Illumina 1 M (set B) and Illumina Omni 2.5 M (set C) chips. We then imputed all remaining CG SNP genotypes available using Impute2 (default parameters) and the various call sets as reference panels. We imputed 315,326 SNPs from set A, 823,570 SNPs and 27,511 indels from set B, and 775,818 SNPs and 27,511 indels from set C. We defined as isolated, an indel with no other indel in the 50 bp flanking regions. We found 23,641 (85.9%) isolated indels and 3,870 (14.1%) non-isolated indels. All these variants were then classified into frequency bins that were derived from the official release of haplotypes on a per continental group basis as defined in Supplementary Table 2 . Then, for each continental group and frequency bin separately, we measured the squared Pearson correlation coefficient between the true (CG derived) and the imputed dosages, ranging from 0 in case of completely wrong imputation to 1 in the case of a perfect imputation. Note that a genotype dosage is the expected number of copies of non-reference alleles; being 0, 1 or 2 in the case of a known genotype and ranging from 0 to 2 in the case of an imputed genotype. Indels in the phase 1 1000GP haplotypes were filtered at 1% which explains why there are no results for very low-frequency indels in Fig. 2d . How to cite this article: Delaneau, O. et al. Integrating sequence and array data to create an improved 1000 Genomes Project haplotype reference panel. Nat. Commun. 5:3934 doi: 10.1038/ncomms4934 (2014).